Quantum replication at the Heisenberg limit No process in nature can perfectly clone an arbitrary quantum state. But is it possible to engineer processes that replicate quantum information with vanishingly small error? Here we demonstrate the possibility of probabilistic super-replication phenomena where N equally prepared quantum clocks are transformed into a much larger number of M nearly perfect replicas, with an error that rapidly vanishes whenever M is small compared with N 2 . The quadratic replication rate is the ultimate limit imposed by quantum mechanics to the proliferation of information and is fundamentally linked with the Heisenberg limit of quantum metrology. No physical process can copy arbitrary quantum states on demand [1] , [2] ; if such a process existed, we could build a device that distinguishes quantum states with arbitrary precision, violating the uncertainty principle and enabling faster-than-light communication [3] . Probabilistic processes like stimulated emission, however, seem to evade this restriction. In Einstein’s treatment of stimulated emission [4] , an excited atom interacting with a polarized photon is expected to produce sometimes a second photon with the same polarization, effectively delivering a perfect clone. True that some other times the atom will spontaneously emit a photon of random polarization, but still, when stimulated emission occurs, a perfect clone has been produced. If we had on our side a quantum version of Maxwell demon, who separates the photons produced by stimulated emission from those produced by spontaneous emission, we would be able to generate any desired number of clones with a non-zero probability. Unfortunately, our imaginary helper is not allowed by the laws of quantum mechanics, even with tiny probability, knowing whether or not stimulated emission took place would lead to a violation of the no-signalling principle (incidentally, this observation should be taken as a reminder that Einstein’s treatment is just an approximation, whereas in the actual quantum dynamics stimulated and spontaneous emission happen in a coherent superposition). However, nothing forbids that other probabilistic processes, akin to spontaneous emission, could proliferate quantum information beyond any previously conceived limit. This possibility raises new fundamental questions: is it possible to engineer a process that duplicates a beam of N equally prepared particles, producing a beam of 2 N almost perfect clones? What is the ultimate rate at which quantum information proliferate without significant errors? Here we answer both questions: although it is impossible to duplicate arbitrary quantum states, we devise a probabilistic mechanism that transforms an input beam of N particles, equally prepared in a state = e − itH generated by time evolution, into an output beam of magnified intensity, consisting of an overwhelming number M of nearly perfect clones with a small error that vanishes rapidly whenever M is small compared with N 2 . We name this new phenomenon super-replication and show that it is intrinsically probabilistic, by proving that deterministic processes can only produce a negligible number of nearly perfect replicas. For example, for 100 linearly polarized photons, super-replication allows one to produce 1,000 replicas with fidelity 99.9%, whereas the best deterministic process can only achieve fidelity 57%. In addition, we show that no physical process, deterministic or not, can proliferate quantum information at a rate larger than quadratic; any attempt to replicate quantum information beyond this limit is doomed to produce a joint output that has vanishing fidelity with the desired state. To explain the roots of this fundamental limitation, we establish a deep link between quantum cloning and the precision limits of quantum metrology [5] , [6] , [7] , [8] , [9] , [10] , [11] , showing that the Heisenberg limit (HL) sets the ultimate bound to the replication rate of probabilistic processes, while the standard quantum limit (SQL) sets the corresponding bound in the deterministic regime. The SQL for information replication Optimal cloning is a fundamental primitive in quantum information [12] , [13] , [14] . Its goal is to transform N input copies of a quantum state , randomly drawn from a set { } x ∈ X , into M approximate copies that are as faithful as possible. The simplest figure of merit here is the fidelity F N → M between the M -particle state produced by the process and M exact copies of the desired state, evaluated on the worst-case input state. Inspired by information theory, we now consider a sequence of cloning processes that transform N input copies into M = M ( N ) approximate copies and we say that the replication is reliable if the replication error vanishes in the limit of large N . As an error measure, we use the infidelity e N → M :=1− F N → M . Here the crucial question is how large can M grow as a function of N in a reliable replication process? To answer the question, we introduce the notion of replication rate, saying that a replication process has rate α if the number of extra copies scales like N α . We say that a rate is achievable if there exists a sequence of reliable replication processes with that rate. We will now see that the achievable replication rates are determined by the precision limits of quantum metrology. Our first key result in this direction is a SQL for quantum replication: No deterministic process can reliably replicate a continuous set of quantum states at a rate larger than 1. In other words, deterministic processes can only embezzle from nature a negligible number of extra copies. The derivation of the SQL for quantum replication is based on the SQL for quantum metrology [15] , applied to an arbitrary curve of states { | t ∈ (− ε , ε )} contained in the set of states that we are trying to clone. A sketch of proof is as follows: the SQL states that the variance in the estimation of t from N copies is lower bounded by , for a constant c that can be set to c =1 with a suitable choice of parametrization. Now, suppose that there is a sequence of reliable deterministic processes with rate α . The N th process will produce an M -particle output state , where M ≥ N + aN α for some constant a >0, approaching the ideal target in the large N limit. For simplicity, let us assume that the trace distance between and vanishes as O ( M − β ) for some exponent β ≥1 (for sets of states of the form , this assumption is lifted in Supplementary Note 1 ). Now, if two states are close, so is the variance in the estimation of t from these two states: for every fixed estimation strategy, we have the bound , where is the variance in the estimation of t from , V M , t is the variance in the estimation of t from M copies and γ >0 is a suitable constant. However, applying a deterministic transformation cannot reduce the variance of the optimal estimation strategy, denoted by . Hence, we have the bound . Choosing the best estimation strategy, we then obtain . Now, since the SQL is asymptotically achievable by a suitable strategy ( cf . Methods), for large N the bound becomes 1/ N ≤1/( N + aN α )+γ( N + aN α ) − β , up to terms that are negligible with respect to N −1 . Clearly, this implies α ≤1 because otherwise we would have a contradiction for large N . This establishes the SQL for quantum replication. As a by-product of the derivation, we also have that no deterministic process can replicate information with error vanishing faster than N −4 . Indeed, by Taylor expanding on the right hand side of the inequality 1/ N ≤1/( N + aN α )+ γ ( N + aN α ) − β , we obtain the condition β ≤2− α , which implies β ≤2. Using the relation between fidelity and trace distance [16] , this means that the replication error is lower bounded as e N → M ≥ O ( N −4 ). In other words, for a reliable replication process the error cannot vanish faster than a low-degree polynomial. The SQL limits not only deterministic replication but also some instances of probabilistic replication; for example, probabilistic cloning has no advantage for arbitrary pure states (this fact was observed in [17] for 1-to- M cloning, but the argument can be easily extended to N -to- M cloning). More generally, it is easy to see that if the set of states { } has strong symmetries, probabilistic processes do not lead to any improvement ( cf. Methods). A sketch of the argument is the following: any probabilistic process can be decomposed into the application of a filter—that transforms an input state into the output state for some suitable operator M yes —followed by a deterministic process. Now, if the set of states has strong symmetries, the optimal operator M yes is forced to be equal to the identity, and the probabilistic process becomes equivalent to a deterministic one. This is the case for cloning of arbitrary pure states [18] , coherent states [19] or coherent spin states [20] , where the replication rates are bound to satisfy the SQL. The HL for information replication We now restrict our attention to the replication of states of the form , t ∈ , where H = H † is a suitable Hamiltonian. We call these states clock states, as they can be generated through a time evolution obeying the Schrödinger equation. For simplicity, we focus on finite-dimensional quantum systems and we ignore the uninteresting case where H is a multiple of the identity. The main result here is a HL for the probabilistic replication of clock states. To get the result, we first establish a precision limit for probabilistic metrology where one is allowed to take advantage of filters [21] , [22] . Our strategy is to apply the quantum Cramér-Rao bound (CRB) [7] , [23] , [24] to the states emerging from the filter. By explicit calculation (see Supplementary Note 2 ), we bound the variance at a given point t as where . This innocent-looking application of the CRB leads immediately to a surprise: optimizing over all filters M yes , the right hand side of equation (1) can be made arbitrarily small, suggesting the possibility of unlimited precision ( cf . Methods). Note, however, that to attain the equality in equation (1), one should adapt the choice of filter to the value of t , the unknown parameter that one is trying to estimate. In practice, this is not a realistic scenario. In the case of periodic evolution, a more realistic setting is to have t distributed according to a uniform prior p ( t ) over the period. In this case, the precision that can be achieved on average is still limited: denoting by the expected variance when the particles pass the filter, in Supplementary Note 3 we prove the bound where E max ( E min ) is the maximum (minimum) eigenvalue of the energy such that | ψ has non-zero overlap with the corresponding eigenspace. We note that ( E max − E min ) 2 /4 is equal to the maximum of the variance of H over all possible states | ϕ contained in the subspace generated by the input states { }. Such maximum is achieved by the ‘NOON state’ , where | E max (| E min ) is an eigenstate of H corresponding to the eigenvalues E max ( E min ). Since these states are the best states for deterministic metrology [25] , our result implies that the best strategy for probabilistic metrology with uniform prior consists just in using a filter that generates the NOON state, and then applying the optimal deterministic estimation strategy. Up to a small correction, the same result of equation (2) can be obtained when the evolution is non-periodic, by approximating the uniform distribution with a Gaussian with large variance ( cf . Supplementary Note 4 ). When N identical copies of are available, equation (2) gives the Heisenberg scaling Equipped with this bound, we can now derive the HL for quantum replication; no physical process can reliably replicate a set of clock states at a rate larger than 2. Here is a sketch of the proof: the filter transforms the product state into the entangled state . For this state, equation (3) gives the bound with c =( E max − E min ) −2 + ε ( ε =0 in the case of periodic evolution). Now, suppose that there exists a sequence of probabilistic processes with replication rate α >1, and suppose that the N th process in the sequence produces M ≥ N + aN α approximate copies, with a trace distance from the ideal target vanishing asymptotically as O (1/ M β ), β ≥1 (this assumption is lifted in Supplementary Note 5 ). Then, the variance of the estimation from the output state —denoted by —will be close to the variance of the estimation from ⊗ M : for every t , we will have , for some constant γ independent of t . Taking the average variance over the uniform prior p ( t ), we obtain the relation , where and V M , p are the averages of and V M , t , respectively. By definition, the average variance V M , p is lower bounded by the SQL and the bound is attained in the large M limit by choosing a suitable measurement ( cf . Methods). Hence, by Taylor expanding the terms in M and keeping the leading order terms, we obtain cN −2 ≤4 N − α + O ( N − α ), which implies α ≤2. Note that here β disappeared from the equation as there is no upper bound on β , in principle the error can vanish faster than any polynomial! The HL leaves lots of room for replicating quantum information: for every rate 1< α <2, one has the chance not only to duplicate the input copies but also to produce an overwhelming number of replicas, with an error that vanish faster than any polynomial. In the next paragraph, we will exhibit explicit protocols that have all these features. Our protocols are necessarily probabilistic, as a consequence of the SQL, which constrains deterministic processes to produce a negligible number of extra replicas. Probabilistic super-replication Here we show that clock states can be reliably replicated at any rate allowed by the HL. When the rate is larger than (or equal to) 1, we call the process super-replication to emphasize the fact that it beats the SQL. The key idea to achieve super-replication is to devise a filter that modulates the Fourier amplitudes of the wavefunction in a way that enhances the replication performances to the maximum rate allowed by quantum mechanics. To move to the Fourier picture, we express the input states as , where Spec( H ) denotes the spectrum of the Hamiltonian, is an eigenvector of H with eigenvalue E and p E is the probability that a measurement of the energy gives outcome E . When N identical copies are given, the joint state can be expressed as where H ( N ) = is the total Hamiltonian ( H i denoting the operator H acting on the i th system), | N , E is an eigenvector of H ( N ) for the eigenvalue E and p N , E is the probability that a measurement of the total energy gives outcome E . Choosing a filter M yes that is diagonal in the energy eigenbasis, we can modulate the Fourier amplitudes of the state (4) in any way we like. Of course, since we aim at producing M perfect copies, the natural choice is to replace N with M in the probability distribution p N , E . However, the spectrum of H ( N ) may be not be contained in the spectrum of H ( M ) and in general one needs to shift the energy values by a suitable amount δ E 0 ≈( M − N ) ψ | H | ψ (see Supplementary Note 6 ). With this choice, the state after the filter is projected to the entangled state . The state will now act as a quantum programme, containing the instructions that will be used by a deterministic quantum device to generate M approximate clones. For this purpose, we use a device that coherently transforms each eigenstate | N , E into the corresponding eigenstate | M , E +δ E 0 , thus producing the state . It is not hard to see that the state has high fidelity with the desired state for every replication rate allowed by the HL. Precisely, for large enough N one has the bound where K is the number of energy levels E such that p E ≠0 and p min =min{ p E : p E ≠0} (see Supplementary Note 7 for the proof). Equation (5) shows that the fidelity approaches 1 faster than any polynomial whenever M is of order N α with α <2, that is, whenever the replication rate satisfies the HL. A strong converse can be proven: every process replicating quantum states at a rate higher than 2 must have vanishing fidelity in the limit of large N , as showed in Supplementary Note 5 . Thanks to our filter, we have been able to embezzle from nature a large number of replicas. The improvement is striking if one compares it with the performances of standard cloning processes. Let us illustrate this fact for the replication of linear polarization states =cos t +sin t . In this case, the best deterministic process is the phase-covariant cloner of [26] , and its fidelity is in the asymptotic limit of large N and M . In agreement with our SQL, the fidelity vanishes whenever M is of order N 1+ ε , ε >0. As we proved in general, deterministic processes can only produce a number of extra replicas that is a negligible fraction of the number of input photons. In stark contrast, for N =100 input photons, our filter can produce M =1,000 approximate copies with fidelity F prob =0.9986, whereas the fidelity of the optimal deterministic cloner is only F det =0.5739. In the example of linearly polarized photons, our filter is provenly optimal, as it coincides with the optimal probabilistic cloner of [17] . Quite surprisingly, the possibility of super-replication was not recognized in [17] where the advantage of probabilistic processing was conjectured to be only of the order of one percent. The different features of replication processes at the HL and at the SQL are illustrated in Fig. 1 in the case of linearly polarized photons. 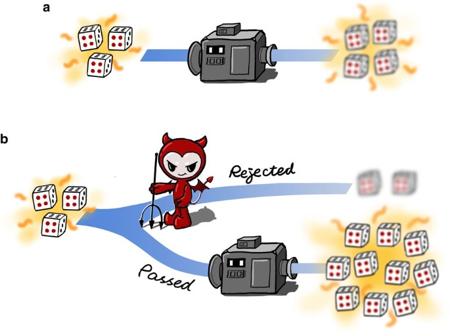Figure 1: The advantages of probabilistic super-replication. (a) Every deterministic process is constrained by the SQL: the number of clones that can be produced reliably fromNinput copies is of orderNand the fidelity of the clones cannot approach 1 faster than the inverse of a polynomial of degree 4. (b) Super-replication at the HL: the cloning performances can be dramatically increased by a probabilistic filter, depicted here as a ‘quantum Maxwell demon’ that separates two branches of the wavefunction. In the successful branch, any number of clones of orderN2−εcan be produced with fidelity approaching 1 faster than any polynomial. Figure 1: The advantages of probabilistic super-replication. ( a ) Every deterministic process is constrained by the SQL: the number of clones that can be produced reliably from N input copies is of order N and the fidelity of the clones cannot approach 1 faster than the inverse of a polynomial of degree 4. ( b ) Super-replication at the HL: the cloning performances can be dramatically increased by a probabilistic filter, depicted here as a ‘quantum Maxwell demon’ that separates two branches of the wavefunction. In the successful branch, any number of clones of order N 2− ε can be produced with fidelity approaching 1 faster than any polynomial. Full size image The advantage of the filter is clear also in the non-asymptotic setting: a plot comparing the performances of replication with and without the filter in the case N =20 is presented in Fig. 2 . 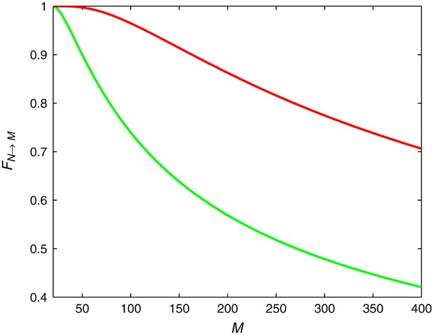Figure 2: Replication of linearly polarized photons. The fidelity of the best cloning processes for linearly polarized photons=cost|V+sint|His plotted here forN=20 input copies, with the numberMof output clones ranging from 20 to 400. The red (green) line refers to optimal cloning with (without) filter. Figure 2: Replication of linearly polarized photons. The fidelity of the best cloning processes for linearly polarized photons =cos t | V +sin t | H is plotted here for N =20 input copies, with the number M of output clones ranging from 20 to 400. The red (green) line refers to optimal cloning with (without) filter. Full size image What makes the improvement even more dramatic is that the quality of the replicas is measured by the global fidelity between the output state and the desired joint state of M perfect copies, which is much smaller than the fidelity that each single copy has with the state . Maximizing the probability of success The dazzling performances of super-replication come at a price: the probability that the input systems pass the filter has to decay with N . Indeed, in Supplementary Note 1 we already showed a strong converse of the SQL: every deterministic process producing replicas at a rate higher than the SQL must have vanishing fidelity. For our filter, the probability of super-replication at rate α >1 decreases exponentially fast as p yes [ N → M ]≤ e − kN for a suitable constant k >0 independent of α (see Supplementary Note 8 ). One may ask whether there are ways to achieve super-replication with a larger success probability. It turns out that the answer is yes. In Supplementary Note 9 , we show that a process producing M ≤ O ( N ) replicas can have a success probability p yes [ N → M ] going to zero as 1/ N δ for every desired δ >0. Most importantly, for a super-replication process with rate α =1+ ε , ε >0, we show how to increase the success probability to p yes [ N → M ]≥ e − Nδ for every desired exponent δ > ε . However, no further improvement is possible below the critical value δ c = ε ; any process with success probability scaling as p yes [ N → M ]= ae − bNδ , δ < ε , a , b >0 must have vanishing fidelity in the asymptotic limit, as observed in Supplementary Note 1 . These results identify the optimal exponent for the decay of the success probability in a super-replication process, pinning down the trade-off between the replication rate and success probability. Interestingly, the choice between the advantage of a high replication rate and that of a unit success probability can be always delayed to the very last moment. Indeed, it is easy to see that asymptotically the best deterministic replication process is just given by the coherent transformation that we used in our protocol. Hence, an alternative way to achieve super-replication is to apply first the best deterministic process and later to modulate the Fourier amplitudes of the wavefunction using a probabilistic filter. Many-worlds fairness Super-replication can be achieved not only for one-parameter families of clock states but also for different manifolds of states, including the manifold of all maximally entangled states of two identical systems. However, super-replication is not a generic feature. As we already mentioned, if one tries to copy an arbitrary—as opposed to linear—polarization state, then no filter is going to help; the performances with filter are equal to the performances without filter. More generally, for generic quantum systems, no probabilistic filter can make an arbitrary quantum state more copiable. This property is quite compelling when considered from the angle of the many-worlds interpretation of quantum mechanics [27] because it states that no-branch of the wavefunction of the universe offers an advantage over the others in replicating the information contained in a completely unknown state. Regarding different branches as ‘different worlds’, we can formulate this as a fundamental principle, which we name many-worlds fairness: the maximum rate at which arbitrary information can proliferate is the same in all possible worlds. Many world fairness rules out quantum mechanics on real Hilbert spaces [28] , an alternative physical theory where photons can have only linear polarizations. Thanks to this observation, one can provide a new answer to the old question‘why are physical systems described by complex—instead of real—Hilbert spaces?’. Traditionally, the standard answer has been to invoke local tomography, the property that one can completely identify a mixed state from the statistics of local measurement on the components. However, one may consider this as an ad hoc requirement [29] , and, in fact, there are even reasons to prefer real quantum mechanics to its complex version, as it was recently pointed out by Wootters [30] . Balancing this fact, many-world fairness offers a new reason (other that the usual local tomography) in favour of complex quantum mechanics. Super-replication has been introduced here from a theoretical point of view. But is it possible to implement it experimentally? Luckily, very recently there have been experimental breakthroughs on the closely related topic of probabilistic amplification of coherent states of light [31] , [32] , [33] , [34] , [35] . Although the translation to our case is not immediate, we suggest that super-replication of linearly polarized photons could be achieved through a suitable sequence of amplitude-damping channels, which for the polarization play the role of the photon subtraction for coherent states. An alternative approach is to first encode the state of the input copies into a coherent state via matter-light teleportation [36] , amplify the coherent state in a probabilistic fashion, and then teleport back. This scheme provides a new application of the existing experimental schemes for coherent state amplification, making them the building block for the replication of quantum information at the HL. Finally, a third avenue towards implementing super-replication would be through stimulated emission, combined with a suitable monitoring of the emitting atoms. Simulated emission has been discussed extensively in connection with deterministic cloning [37] , [38] , [39] , but its potential for implementing probabilistic processes is still unexplored. In relation to the existing literature, it is interesting to comment on the relation between our results and previous works on probabilistic cloning and probabilistic estimation. The idea that in some situations even non-orthogonal states can be copied perfectly using a probabilistic device was first introduced by Duan and Guo [40] who showed that a set of pure quantum states can be copied perfectly if and only if they are linearly independent. This means that for a single photon, one can perfectly copy two polarization states, while for N photons one can copy at most N +1 states. Subsequent works [17] , [41] , [42] showed that probabilistic devices can improve the performances of approximate cloning for continuous sets of states, leading to nearly ideal performances in the case of coherent states with fixed amplitude. The nearly perfect cloning of coherent states may lead one to believe that in general there is no limit to the amount of clones that can be produced probabilistically. Contrarily to this intuition, we have proven here that for finite quantum systems, the HL sets the ultimate bound M = O ( N 2 ) to the number of clones that can be produced reliably. Moreover, we have shown that for arbitrary one-parameter families of states, any replication rate allowed by the HL can be achieved and we identified exactly the exponent at which the probability of success has to decay. Finally, the relation between cloning and estimation has been extensively investigated in the literature [43] , [44] , [45] , [46] , [47] in terms of single-copy fidelities. However, none of the approaches proposed so far was suitable to derive limits on the asymptotic replication rates, nor to connect the latter with quantum metrology. Recently, it has been observed that the precision of quantum estimation can be improved using probabilistic strategies [21] , [22] where depending on the outcome of the filter, one can decide to abstain from estimating the parameter. The mechanism of abstention can sometimes boost the precision from the SQL 1/ N to the HL 1/ N 2 . The connection between these results and super-replication is made clear by our approach: the fact that a probabilistic filter can improve estimation until the HL implies that N 2 , rather than N , is the upper bound for the replication rate of the states = e − itH . However, there is an important catch: the filter that achieves replication at the HL is not the same filter that achieves estimation at the HL. In fact, if we were to use the same filter needed in [21] , [22] , we would not be able to reduce the error down to zero. Decomposition of quantum instruments To describe the most general probabilistic processes allowed by quantum mechanics, we use the framework of quantum instruments [48] , [49] , [50] . A quantum instrument with input (output) Hilbert space ( ) is a collection of completely positive (CP), trace non-increasing linear maps { } j ∈ Y , where each map transforms density matrices on into (sub-normalized) density matrices on . If the input system is prepared in the density matrix ρ , the probability that outcome j is p ( j | ρ )= Tr [ (ρ)]. Conditionally, to the occurrence of outcome j , the state of the output system is . We note an elementary fact about quantum instruments: any quantum instrument can be decomposed into a pure measurement on the input system followed by quantum channel depending on the outcome. By ‘pure measurement on the input system’, we mean a quantum instrument { } j ∈ Y of the special form for some operator M j on . By ‘quantum channel’, we mean a trace-preserving CP map C j , transforming density matrices on into (normalized) density matrices on . In formula, our claim is that every CP map can be decomposed as The proof is as follows: let be the adjoint of the map , defined by for every operator A and for every density matrix ρ . Define the operator and the map by the relation , where is the inverse of M j on its support. If M j is invertible, then := is trace preserving: In this case, by definition we have for every ρ . If M j is not invertible, we can define the trace-preserving map ( ρ ):= ( ρ )+ P ⊥ ρP ⊥ , where P ⊥ is the projector on the kernel of M j . Again, the definition implies for every state ρ . For the purposes of this paper, it is enough to consider measurements with two outcomes (yes,no), referred to as filters. The filter induces a bifurcation of the wavefunction and selects one particular branch, corresponding to the successful outcome yes. Symmetry constraints on probabilistic cloning Consider a quantum cloning problem where the set of states { } has a group of symmetries, denoted by G. This means that, for every unitary operator U g representing the action of a symmetry transformation in the group, one has { U g } x ∈ X ={ } x ∈ X . A probabilistic cloner is described by a quantum instrument { , } from the space of N copies to that of M copies, where the CP maps and correspond to the successful and unsuccessful instances, respectively. Conditional to the successful outcome, the fidelity of the output state with the desired M -copy state is The goal of cloning is to maximize the worst-case fidelity . Because of the symmetry of the set of states, the maximization can be restricted without loss of generality to the set of covariant CP maps, that is, of CP maps satisfying the relation for every group element g and for every quantum state ρ . The proof is standard and we refer the interested reader to similar proofs provided in the literature, such as those of [51] , [52] for covariant measurements and that of [53] for covariant cloning channels. Let us work out the implication of symmetry, starting from the decomposition = of equation (6). It is easy to see that the covariance of P yes implies the commutation relation , for every group element g . Indeed, using the definition and the covariance of , we have Now, if the group of symmetries is sufficiently large, the action of the unitaries can be irreducible in the subspace containing the input states . When this happens, the Schur’s lemma imposes that the filter M yes be a multiple of the identity, and, therefore . By equation (7), this means that the fidelity achieved by the CP map is the same as the fidelity achieved by the quantum channel . In summary, we have proven the following fact: the maximum of the fidelity over all probabilistic cloners is equal to the maximum of the fidelity over deterministic cloners whenever the action of the unitaries is irreducible in the subspace spanned by the input states { }. This simple observation has several important consequences. A first consequence, noted by Fiurášek [17] , is that the probabilistic processes do not offer any advantage for 1-to- M cloning of arbitrary pure states. Our approach allows to reach the same conclusion in a fairly broader range of cloning problems: in particular, it implies that probabilistic processes offer no advantage in the case of N -to- M cloning of arbitrary pure states [18] , N -to- M cloning of coherent states [19] and spin-coherent states [20] , 1-to- M cloning of two Fourier transformed bases [53] and of all the sets of states considered in [53] , and 1-to- M phase-covariant cloning for qubit states on the equator of the Bloch sphere [26] . Pointwise versus average CRB The CRB is the cornerstone of quantum metrology [5] , [6] , [7] , [8] , [9] , [11] . For a family of clock states = e − itH , it states that the variance in the estimation of t from the state is lower bounded by V t ≥1/ Q t , where Q t :=4( H 2 − H 2 ) is the quantum Fisher information (QFI). The equality in the CRB can be achieved if one adapts the estimation strategy to the value of t . This can be done in an asymptotic scenario when one is given a large number of copies of and uses a fraction of them to obtain a rough estimate of t ( [54] ). However, if instead of having N copies one has a single N -particle entangled state, the CRB may not give an achievable lower bound. For example, Hayashi [55] showed that the CRB for phase estimation predicts the correct scaling c / N 2 , but with a constant c that is not achievable. In the case of probabilistic metrology, the issue about the achievability of the CRB appears in a more dramatic way: if we allow one to adapt also the choice of the filter M yes to the value of t , then the CRB promises unlimited precision. It is instructive to see how this phenomenon can happen. For a given t 0 , choose a parametrization where H =0 (this can always be done by redefining H as H ′= H − H ). Then, define the vector which by construction satisfies . Now, choose the filter operator The filter does not change the state : However, it amplifies the time derivative at t 0 : where in the second line we used the explicit expression along with the observation that . As a result, the probabilistic QFI at t 0 , defined as the QFI associated to the states , satisfies This equation means that, whenever the original QFI is non-zero at a specific value t 0 , the probabilistic QFI can be made arbitrarily large with a suitable choice of ε . This fact, combined with the CRB, seems to suggest that one can have unlimited precision. However, such a conclusion is an artifact of the pointwise character of the CRB: the probabilistic estimation scheme shown above has unlimited precision only in an infinitesimally small neighbourhood of t 0 . In light of this observation, for probabilistic metrology, it is more sensible to choose the filter M yes independent of t , to assign a prior p ( t ) to the unknown parameter and to minimize the expected variance. Note that, since the estimate is produced only when the system passes through the filter, the expectation has to be computed with respect to the conditional probability distribution . The expected variance, denoted by , is lower bounded by the inverse of the expected QFI, denoted by in formula The proof of equation (9) is an elementary application of the pointwise quantum CRB and of the Schwartz inequality: Note that the average CRB of equation (9) is just a lower bound and the equality may not be achievable. However, achievability is of no consequence for our arguments about the replication rates. How to cite this article: Chiribella, G. et al. Quantum replication at the Heisenberg limit. Nat. Commun. 4:2915 doi: 10.1038/ncomms3915 (2013).